Single-shot pulse duration monitor for extreme ultraviolet and X-ray free-electron lasers The resolution of ultrafast studies performed at extreme ultraviolet and X-ray free-electron lasers is still limited by shot-to-shot variations of the temporal pulse characteristics. Here we show a versatile single-shot temporal diagnostic tool that allows the determination of the extreme ultraviolet pulse duration and the relative arrival time with respect to an external pump-probe laser pulse. This method is based on time-resolved optical probing of the transient reflectivity change due to linear absorption of the extreme ultraviolet pulse within a solid material. In this work, we present measurements performed at the FLASH free-electron laser. We determine the pulse duration at two distinct wavelengths, yielding (184±14) fs at 41.5 nm and (21±19) fs at 5.5 nm. Furthermore, we demonstrate the feasibility to operate the tool as an online diagnostic by using a 20-nm-thin Si 3 N 4 membrane as target. Our results are supported by detailed numerical and analytical investigations. Extreme ultraviolet (XUV) and X-ray free-electron laser (FEL) sources have taken a central role in science for a broad variety of communities ranging from physicists to biologists and medical scientists. Meanwhile, FELs are operated as large-scale user facilities providing intense XUV and X-ray radiation to study ultrafast dynamics on the nanoscale and within atoms, molecules and solids [1] , [2] , [3] , [4] , [5] , [6] , [7] , [8] , [9] , [10] . One of the great expectations from free-electron lasers is the application of X-ray coherent diffraction imaging to a single molecule within its functional environment [9] . The tailoring of plasma states of matter and the investigation of their evolution at short timescales can also be achieved [10] . High-resolution pump-probe experiments require a precisely characterized FEL pulse and precise synchronization to an external optical pump-probe laser. While so far different schemes for arrival time measurements have been developed [11] , [12] , [13] , [14] , [15] , [16] , [17] , [18] , [19] , [20] , [21] , [22] , [23] , insufficient characterization of the XUV or X-ray FEL pulse duration at the experimental station remains the main handicap of single pass free-electron lasers that rely on self-amplified spontaneous emission (SASE). Direct and indirect techniques for XUV and X-ray pulse duration measurement [22] , [23] , [24] , [25] , [26] , [27] , [28] , [29] , [30] , [31] , [32] and pulse arrival time monitoring [11] , [12] , [13] , [14] , [15] , [16] , [17] , [18] , [19] , [20] , [21] , [22] , [23] are subjects of active research and most are already implemented in the FEL machine environment. In particular for XUV pulses, the experiments must be realized under vacuum conditions. Thus, measuring the pulse duration directly is a complex and invasive endeavour that requires extensive experimental resources. Techniques such as XUV autocorrelation, optical/XUV cross-correlation are not single-shot measurements and require, for example, XUV split-and-delay optics and time-of-flight spectrometers [24] , [25] , [26] . The light-field streaking method requires a sophisticated set-up for generating strong single-cycle terahertz fields [22] or additional dedicated FEL infrastructure [23] . Furthermore, these techniques are limited to a certain range of wavelengths and pulse durations, as they rely on atomic transition levels in gaseous targets. In the case of timing diagnostic tools, a disadvantage of many methods is that the spatial distance to the actual experiment introduces an additional timing uncertainty. One category of diagnostics is designed only to measure the arrival time of the electron bunches with respect to the pump-probe laser [11] , [12] , [13] . This has the disadvantage that the path length drift of the photon beamlines is omitted. Additionally, the synchronization drift of the pump-probe laser to the master clock of the accelerator is also not considered. Another category of diagnostics is to directly measure the timing of the XUV pulses [14] , [15] , [16] , [17] , [18] , [19] , [20] , [21] , [22] , [23] . Most of those measurements, such as X-ray optical cross-correlators, are highly invasive and cannot be performed simultaneously with other pump-probe experiments. In this work, we report a concept that allows for a single-shot FEL pulse duration measurement in combination with arrival time monitoring directly at the experimental station. The technique is applicable for pulse durations from a few femtoseconds to a few hundreds of femtoseconds in a wide range of soft X-ray and XUV wavelengths. Our proposed method is based on XUV/optical cross-correlation using solid-state targets. It can be applied directly at the experimental station with a considerably less complex experimental set-up compared with the methods described above. Furthermore, we show a solution allowing the XUV beam to be reused for a simultaneous pump-probe experiment. This novel temporal diagnostic tool can also be applied at X-ray FELs, as recently demonstrated for arrival time monitoring [20] , [21] . Experimental set-up The experimental set-up is illustrated in Fig. 1a . An intense XUV pulse from the free-electron laser FLASH is absorbed at the surface of a solid target, which is illuminated by a largely collimated near-infrared probe laser pulse. Using a microscope objective, the transmitted infrared light from the sample surface is imaged onto a CCD. Owing to the XUV absorption, a high electron density is produced within the conduction band of the sample surface. The resulting ultrafast change of the optical transmission is related to the absorbed FEL fluence und thus follows its intensity envelope. The non-collinear beam geometry between FEL and probe laser allows for single-shot spatio-temporal decoding. As depicted in Fig. 1a , the spatial coordinates, x 0 and x 1 , of the incident XUV pulse correspond to different arrival times, t 0 and t 1 , of the tilted FEL wavefront. Hence, the spatial x axis in the image represents the cross-correlation between the temporal evolution of the plasma transmission and the intensity of the probe laser. We performed detailed theoretical studies to investigate the relationship between the FEL intensity envelope and the measured transmission change. As a result, we show that the FEL pulse duration can be extracted. Our measurements are performed at the wavelengths of 41.5 and 5.5 nm. 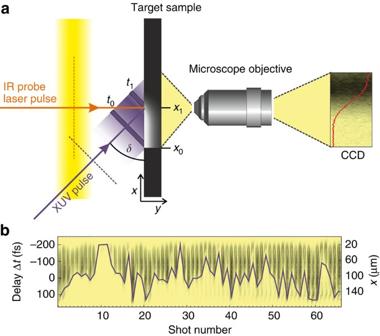Figure 1: Single-shot pulse duration and arrival time measurements. (a) Schematic of the experimental set-up. The XUV pulse with a beam diameter of ~100 μm FWHM is incident under an angleδwith respect to the sample surface (material: SiO2, Si3N4). Within a single shot, different temporal partst0,t1of the XUV wavefront are absorbed at different spatial positionsx0,x1on the sample, providing a spatio-temporal decoding. A largely collimated near-infrared pulse under normal incidence is used to probe the optical transmission change within the surface during the absorption. The transmitted light is imaged onto a CCD. (b) Series of single shots recorded with 10 Hz acquisition rate. The black shading represents the increased optical opacity due to an increased electron density within the conduction band of the sample surface. The spatial position of the transient bottom edge on thexaxis is dependent on the relative arrival time between the probe laser and the FEL pulse. The solid line indicates the extracted arrival time. Figure 1: Single-shot pulse duration and arrival time measurements. ( a ) Schematic of the experimental set-up. The XUV pulse with a beam diameter of ~100 μm FWHM is incident under an angle δ with respect to the sample surface (material: SiO 2 , Si 3 N 4 ). Within a single shot, different temporal parts t 0 , t 1 of the XUV wavefront are absorbed at different spatial positions x 0 , x 1 on the sample, providing a spatio-temporal decoding. A largely collimated near-infrared pulse under normal incidence is used to probe the optical transmission change within the surface during the absorption. The transmitted light is imaged onto a CCD. ( b ) Series of single shots recorded with 10 Hz acquisition rate. The black shading represents the increased optical opacity due to an increased electron density within the conduction band of the sample surface. The spatial position of the transient bottom edge on the x axis is dependent on the relative arrival time between the probe laser and the FEL pulse. The solid line indicates the extracted arrival time. Full size image Ultrafast ionization processes The irradiation of dielectrics with ultrashort XUV and X-ray laser pulses causes photoionization of electrons from bound states (deep shells and valence band) to high-energy states of the conduction band, producing energetic free electrons. A dedicated Monte-Carlo simulation tool [33] , [34] , [35] , [36] , [37] was applied to study the relaxation of the photoexcited electronic subsystem within a solid SiO 2 target irradiated with an 80-fs Gaussian XUV pulse. Typical simulation times were of the order of a few hundreds of femtoseconds. With this method that follows individual electrons and holes event-by-event, the density and the distribution function of the electrons within the conduction band and of the holes within the valence band were obtained. The following processes were considered: photoabsorption by bound and excited electrons, secondary impact ionizations by free electrons, elastic scattering of electrons, and Auger decay of the deep shells. The primary photoionization, impact ionization and Auger-decays lead to the increase of the electron density in the conduction band that occurs during and shortly after the laser pulse (for details see Methods section). For XUV photon energies below 1 keV ( λ FEL >1.23 nm), the electron density can be assumed to directly follow the integrated laser intensity envelope on the timescale of sub-femtoseconds to a few femtoseconds. With increasing photon energy, the contribution of secondary processes such as impact ionization and Auger processes becomes dominant and these cascades themselves last longer. Owing to the longer electron rise time, the resolution is reduced to the few-10-fs scale [37] . In Fig. 2a , the dependence of the electron density, , on the FEL fluence, F , is calculated for different XUV wavelengths, 5.5 nm (black), 13.6 nm (blue) and 41.5 nm (red). Apparently, the electron density grows linearly with the photon flux, for all studied FEL photon energies, , within F <0.05 J cm −2 . According to previous theoretical results [34] , the number of electrons that is produced by one photon can be determined by the ratio between photon energy and the effective energy gap ( EEG ) of the material, . This allows us to find an analytical expression for the temporally varying electron density distribution, , along the FEL propagation axis, y , within the sample surface. 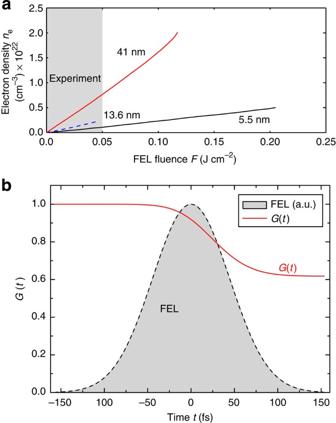Figure 2: Analysis of the plasma gating process. (a) Electron density,ne, within the conduction band of fused silica as a function of the fluence of an 80-fs XUV pulse, calculated using a dedicated Monte-Carlo simulation for different wavelengths, 41.5 nm (red line), 13.6 nm (blue dashed line) and 5.5 nm (black line). The grey shaded region represents the linear absorption regime for fluences below 0.05 Jcm−2. The experimental conditions were chosen accordingly. (b) Calculated transmissionG(t) (red) generated by the temporal plasma evolution of an absorbed Gaussian FEL pulse with 105 fs pulse duration (grey). For each individual moment in time, the absorbed FEL intensity follows Beer’s absorption law: Figure 2: Analysis of the plasma gating process. ( a ) Electron density, n e , within the conduction band of fused silica as a function of the fluence of an 80-fs XUV pulse, calculated using a dedicated Monte-Carlo simulation for different wavelengths, 41.5 nm (red line), 13.6 nm (blue dashed line) and 5.5 nm (black line). The grey shaded region represents the linear absorption regime for fluences below 0.05 Jcm −2 . The experimental conditions were chosen accordingly. ( b ) Calculated transmission G ( t ) (red) generated by the temporal plasma evolution of an absorbed Gaussian FEL pulse with 105 fs pulse duration (grey). Full size image The FEL pulse penetrates into the material by a distance 1/ along y . The XUV absorption coefficient, , can be taken from [38] . The corresponding XUV photon flux is proportional to the temporally integrated intensity: Here we assume that the initial flux is zero, . From this distribution, we calculate the electron density produced by photoionization: According to equation (5), we assume that the electron density instantaneously follows the integrated FEL intensity envelope. Plasma gating Optical radiation from the probe laser pulse is being reflected and absorbed by the plasma electrons. Hence, an optical pulse travelling through the XUV-irradiated region will be gated by the plasma transmission. For electron densities around the critical plasma density, cm −3 at the probe laser wavelength 800 nm, this gating process is to a large extend a result of the ultrafast reflectivity change during the evolution of a thin (sub-wavelength) plasma layer at the sample surface. We calculate the optical properties by applying the Drude model [39] , [40] , [41] to obtain the corresponding complex refractive index profile, , from the electron density in equation (5). The total transmission of the plasma, , is calculated from using the transfer matrix method [42] . Details can be found in the Methods section. The transmitted probe laser intensity represents the cross-correlation, between the gating function, , and a Gaussian probe laser pulse, . It depends on the delay, , between the FEL and the probe pulse as well as on their individual pulse durations. Measuring the cross-correlation using a well-characterized probe laser pulse, , the gating function can be determined. Considering the involved processes described above, we retrieve the intensity envelope of the FEL using a start-to-end simulation, as described in the Methods section. Figure 2b shows the gating function, , generated by the absorption of a Gaussian FEL XUV pulse. When no plasma electrons are present, we normalize , which means that an incoming optical laser pulse will be fully transmitted. The constant reflection at the sample surfaces can be neglected. Correspondingly, when the probe pulse arrives earlier than the FEL pulse, we measure . For a large delay, when the probe laser pulse arrives a few picoseconds later than the FEL pulse, we observe the transmission to remain at a constant level, constant <1. When both pulses temporally overlap, we measure the cross-correlation with a smooth transition from to . The temporal shift of the function is determined by the delay, , between the FEL and the probe laser. Its slope is determined by the FEL and probe laser pulse durations. The ultrafast relaxation of the electron density within 150 fs, which has been observed by other groups using fused silica [43] , [44] , could not be observed. In our experiment, the transmission kept a constant value even for a delay of a few picoseconds. In previous works, the relaxation was associated with the formation of self-trapped excitons, leading to a rapid capture of free carriers [45] . In the present work, the photoionization was triggered by linear absorption of an intense XUV pulse. According to the theoretical calculations, the electron density was up to two orders of magnitudes higher compared with other experiments. We propose that in our experiment a breaking of excitons occurred due to collisions with high energetic electrons within the conduction band. The interpretation is supported by other studies, where it has been shown that excitons, which were formed by low-fluence XUV radiation, can be destroyed by multiphoton absorption of a near-infrared pulse [46] . Pulse duration measurements One such cross-correlation measurement is shown exemplarily in Fig. 3a . The FEL pulse at a wavelength of 5.5 nm was focused onto the sample under an angle of δ =14.2° with respect to the surface. The probe laser pulse propagated through the sample under normal incidence, as explained in the Methods. The achieved spatio-temporal decoding corresponds to a temporal window of 324 fs, according to equation (7) in the Methods section. The image of the transmitted light in Fig. 3a was measured with the laser pulse arriving a few picoseconds later than the FEL pulse. Within this window, no temporal dynamics were observed. Thus, constant plasma conditions can be assumed and the spatial FEL beam profile can be taken as a reference image to correct the signals for spatial features in the FEL profile. 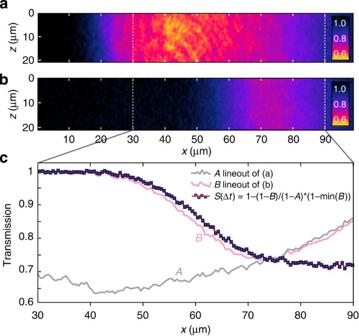Figure 3: Example of the measured transmission change. (a) Transmission along the sample when the optical probe pulse arrives a few picoseconds after the FEL pulse. The reflection change has fully evolved. This reference measurement is used to calibrate the measured signals to the spatial beam profile of the FEL (lineoutA). Along thexaxis, spatio-temporal decoding is achieved according to equation (7). (b) Transmission along the sample when the optical probe pulse and the FEL pulse arrived at the same time. The transient transmission change can be clearly observed (lineoutB), compared with the reference ina. The areas between the white dashed lines indicate the regions of interest for calculating the lineouts. (c) The cross-correlation,S(Δt) (blue rectangles), is obtained by normalization according to the formula in the legend. The signal lineout is inverted by 1−Band normalized to 1−A. The multiplication with 1−min(B) accounts for the constant transmission level after the transient edge, which is around min(B)=0.7 in the presented case. Figure 3b shows a measurement with temporally overlapping laser and FEL pulses. To extract the cross-correlation, , lineouts were calculated from Fig. 3a , as shown in Fig. 3c . Details can be found in the Methods. Figure 3: Example of the measured transmission change. ( a ) Transmission along the sample when the optical probe pulse arrives a few picoseconds after the FEL pulse. The reflection change has fully evolved. This reference measurement is used to calibrate the measured signals to the spatial beam profile of the FEL (lineout A ). Along the x axis, spatio-temporal decoding is achieved according to equation (7). ( b ) Transmission along the sample when the optical probe pulse and the FEL pulse arrived at the same time. The transient transmission change can be clearly observed (lineout B ), compared with the reference in a . The areas between the white dashed lines indicate the regions of interest for calculating the lineouts. ( c ) The cross-correlation, S (Δ t ) (blue rectangles), is obtained by normalization according to the formula in the legend. The signal lineout is inverted by 1− B and normalized to 1 −A . The multiplication with 1−min( B ) accounts for the constant transmission level after the transient edge, which is around min( B )=0.7 in the presented case. Full size image For the determination of the FEL pulse duration, calculations of gating functions were carried out following the mathematics described above. The obtained curves were fitted to the measured data by an optimization routine (see Methods ). The probe laser pulse duration of fs was measured using autocorrelation. For the FEL temporal structure, a Gaussian intensity envelope was assumed. This represents an average over many shots of the lasing of multiple longitudinal modes of SASE FELs [23] , [27] . The FEL operation parameters are described in the Methods section. The electron density, , is determined by the FEL fluence and can be adjusted by varying the FEL energy and the beam diameter. Measured (white rectangles) and fitted (blue line) cross-correlations are shown in Fig. 4 for FEL center wavelengths of 41.5 nm (a) and 5.5 nm (b), respectively. The retrieved pulse durations yield fs at 41.5 nm and fs at 5.5 nm. Uncertainties arise mainly from the probe laser pulse duration and statistical fluctuations of the data points (see Methods ). 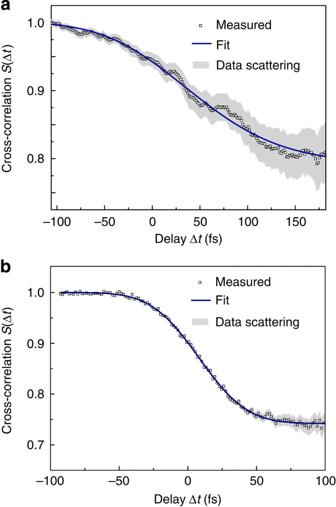Figure 4: Measured cross-correlationsS(Δt) on fused silica targets. (a) Measurement (white rectangles) and fit (blue line) at 41.5 nm FEL wavelength, corresponding to an FEL pulse duration ofτFEL=(184±14) fs. (b) Measurement (white rectangles) and fit (blue line) at 5.5 nm FEL wavelength, corresponding toτFEL=(21±19) fs. The grey data scattering originates from small fluctuations in spatial beam profile features (optical laser and FEL) between two shots taken for the background subtraction. Figure 4: Measured cross-correlations S (Δ t ) on fused silica targets. ( a ) Measurement (white rectangles) and fit (blue line) at 41.5 nm FEL wavelength, corresponding to an FEL pulse duration of τ FEL =(184±14) fs. ( b ) Measurement (white rectangles) and fit (blue line) at 5.5 nm FEL wavelength, corresponding to τ FEL =(21±19) fs. The grey data scattering originates from small fluctuations in spatial beam profile features (optical laser and FEL) between two shots taken for the background subtraction. Full size image To test the applicability of the plasma gating method for online measurements, a feasibility study was conducted using a 20-nm-thin Si 3 N 4 membrane. Thus, the absorption length is reduced compared with the 1-mm-thick fused silica sample. The effective path through the membrane was 98 nm due to the oblique angle of the FEL pulse with respect to the sample surface ( δ =14.2°). The FEL pulse energy of 2.5 μJ was adjusted using the gas attenuator, which is installed in the photon beamline of FLASH. Owing to the lower energy deposition within the thin membrane, the measurement was nondestructive. Measurements on Si 3 N 4 membranes were performed continously on the same sample position and with no visible change in the sample morphology after absorbing a few thousand FEL pulses. In contrast, fused silica samples suffered from radiation damage after ~30 consecutive pulses. Owing to the sufficient residual transmission of FEL energy (~30% at 5.5 nm), the transmitted pulse can be reused for an XUV experiment with simultaneous single-shot characterization of the XUV pulse duration and the relative arrival time to the pump-probe laser. The corresponding single-shot cross-correlation is shown in Fig. 5 , yielding FEL pulses with fs. This value is in agreement with the fused silica measurement and within the error bars. 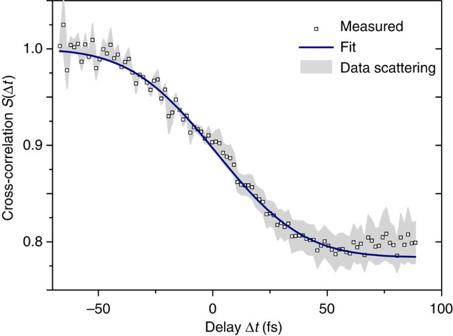Figure 5: Measured cross-correlationS(Δt) on silicon nitride membrane. The sample thickness was 20 nm. The measured (white rectangles) and fitted (blue line) cross-correlation at 5.5 nm FEL wavelength is shown. The retrieved pulse duration isτFEL=(34±19) fs. The grey data scattering originates from small fluctuations in spatial beam profile features (optical laser and FEL) between two shots taken for the background subtraction. The measurements on this sample were nondestructive. This enables the implementation of this method as an online tool for pulse duration and arrival time measurements. Figure 5: Measured cross-correlation S (Δ t ) on silicon nitride membrane. The sample thickness was 20 nm. The measured (white rectangles) and fitted (blue line) cross-correlation at 5.5 nm FEL wavelength is shown. The retrieved pulse duration is τ FEL =(34±19) fs. The grey data scattering originates from small fluctuations in spatial beam profile features (optical laser and FEL) between two shots taken for the background subtraction. The measurements on this sample were nondestructive. This enables the implementation of this method as an online tool for pulse duration and arrival time measurements. Full size image The FEL pulse durations determined by our method are in agreement with the theoretical expectations from accelerator physics [32] . During our experiment, FLASH was operated with a bunch charge of 0.5 nC at 41.5 nm and a charge of 0.25 nC at 5.5 nm. For these high charges, typical electron bunch durations at 41.5 nm are between 140 and 200 fs. The electron bunch durations at 5.5 nm are considerably shorter than 100 fs, but corresponding measurements are not published yet. The correlation between bunch charge and FEL pulse duration is derived from techniques developed earlier, for example, XUV autocorrelation [24] , [25] , XUV/optical cross-correlation [26] , spectral measurements and statistical methods [27] , [28] , [29] , [30] , [31] , [32] , and terahertz streaking [22] , [23] . These complex techniques are not available on demand for direct comparison. Single-shot cross-correlations were measured to determine the FEL pulse duration and arrival time with respect to a ( fs near-infrared probe laser pulse using an ultrafast plasma gating process. The ultrafast change of the electron density is triggered by an FEL XUV pulse on a fused silica sample. The resulting transient change of transmission is convolved with a probe laser pulse of known pulse duration in a spatio-temporal decoding set-up. The obtained single-shot cross-correlations were evaluated using calculations of the optical properties of the plasma, based on linear absorption of the FEL pulse. A dedicated Monte-Carlo simulation was applied to study the ionization process. Exciton breaking due to secondary electron collisions was proposed as the mechanism that prevents ultrafast electron relaxation, which would counteract the plasma buildup. The FEL pulse durations were determined for two distinct wavelengths, yielding fs at 41.5 nm and fs at 5.5 nm. The investigation of complex pulse shapes such as pedestals and multiple pulses is possible by varying the input pulse shapes of the start-to-end fitting procedure. For this purpose, the temporal resolution can be enhanced to the few-femtosecond regime by using sub-10-fs probe pulses and diffraction-limited imaging. For X-ray pulses with photon energies higher than 1 keV, the resolution is limited to the few-10-fs scale because of the longer lasting secondary electron cascades [37] . The method can operate from the XUV to X-ray wavelengths and over a large range of pulse durations as long as the absorption is linear and the duration of the X-ray pulse is longer than the secondary electron cascading. Finally, we also performed measurements using a 20-nm-thin Si 3 N 4 membrane. In this way, we propose a method, which has the potential to simultaneously measure the FEL pulse duration and arrival time, together with the operation of a two-colour pump-probe experiment using ultrashort XUV and near-infrared laser pulses. Experimental set-up The experiment was based on ultrafast microscopy [47] , [48] , [49] , [50] developed for ultrafast studies of optical material properties. The imaging system consisted of a microscope objective (Mitutoyo M Plan APO NIR, NA=0.5) onto a progressive scan charge-coupled device camera (Basler A311f, 659 × 494 pixels). The resolution of the imaging system was calibrated with a periodic micrometre mask (18 cycles per mm). Figure 1a shows the basic interaction scheme in non-collinear geometry. The probe laser pulse from a Ti:sapphire laser amplifier (Coherent Hidra) was aligned under normal incidence to the sample surface. The laser pulse duration was (64±7) fs, the central wavelength was 800 nm. The FEL pulse was aligned under an angle, , with respect to the sample surface, such that different wavefront fractions along the transverse coordinate x reached the sample at different times. The angle of 45° was used for the 41.5-nm measurements and 14.2° during the 5.5 nm measurements, respectively. The arrival time was mapped onto the spatial coordinate, hence the name spatio-temporal decoding. The time axis scale is defined by where c is the vacuum speed of light and is the pixelsize in the image. The shallow angle of 14.2° provided a larger time window than 45°. The measurement was performed at the BL2 beamline at FLASH. The interaction position between XUV FEL pulse and sample surface was out of focus, to adjust the FEL intensity to achieve electron densities around the critical density. The samples used during the experiment were 1-mm-thick fused silica and 20-nm-thin Si 3 N 4 membranes. Free-electron laser operation parameters For the measurements on fused silica targets, the free-electron laser was tuned to two different wavelengths. First measurements were performed at 41.5 nm with average pulse energies of (84±4) μJ. The average electron bunch charge was 0.5 nC. The second wavelength was 5.5 nm with an average pulse energy of around (29±10) μJ. The electron bunch charge was 0.25 nC. The pulse energy was measured with a gas monitor detector [51] . For the study using the Si 3 N 4 membrane, the FEL was tuned to similar parameters, 5.5 nm wavelength and 0.25 nC bunch charge. Physical model and mathematical methods The mathematical description of plasma gating relies on calculating the total optical transmission of the electron plasma for the probe laser wavelength 800 nm. In this context, the temporal evolution of the free-electron density was studied. The applied model [28] , [29] , [30] , [31] accounts for the strongly non-equilibrium conditions during the electron relaxation, as described in the Results section. At the considered simulation times, the radiative decay of electronic vacancies could be neglected because this requires times of typically hundreds of picoseconds to nanoseconds. The formation of self-trapped excitons, which in some materials leads to a fast relaxation of the electron density on the 150 fs scale, could also be neglected. The electron correlation effects resulting from the band structure [52] and Pauli’s principle for excited electrons [34] , [35] , [36] were taken into account. The simulation scheme was as follows. First, the penetration of photons into the material was simulated, according to the intensity envelope of the FEL pulse. For each photon, the penetration depth was calculated, taking into account the attenuation length of the photon in SiO 2 ( [38] ). If this sampled penetration depth lay within the simulation box, the photon was considered as absorbed and its energy was transferred to a randomly chosen electron. The probabilities of the photoabsorption by different shells were taken from the corresponding attenuation lengths [38] . Only single photoabsorptions were considered at the wavelengths of 5.5 nm, 13.6 nm and 41.5 nm and pulse energies of 40 μJ, 6 μJ and 20 μJ, correspondingly [35] . For the fluences studied here, nonlinear effects are negligible, and the temporally resolved free-electron density scaled linearly with the fluence, as it can be seen in Fig. 2a . For evaluating the optical properties, the temporal evolution of the electron density, , was calculated according to equation (5). The thickness of the plasma layer is thus ~20 nm at 41.5 nm and 144 nm at 5.5 nm wavelength. The gating function, , is the total transmission for each point in time of the 800-nm probe laser through the plasma. It was numerically calculated using the transfer matrix method for wave propagation in stratified media [42] . To this end, the exponentially decaying gradient of the electron density was subdivided into thin finite layers with thickness . The complex dielectric constant of each layer was determined from the Drude model [39] , [40] , [41] using the dielectric function, , and the damping factor, , which could be estimated from [39] , [41] . The total transmission of this layered structure was calculated from the resulting transfer matrix, taking into account reflection, transmission, absorption and interference. The obtained gating function, , is used to calculate the cross-correlation with the probe laser pulse (equation (1)) to assess the FEL pulse duration. Deviations of the pulse duration due to uncertainties of the assumed refractive index profiles were within the error bars, as mentioned below. Data analysis The background-corrected images were sorted in two categories, reference images and signal images. The reference images of the evolved plasma were measured with a temporal delay of a few picoseconds between FEL pulse (early) and probe laser pulse (late) to take into account the spatial FEL beam profile as shown in Fig. 3a . The signal images were measured at shorter delays where both pulses overlapped temporally ( Fig. 3b ). Both images were spatially aligned to compensate for the shot-to-shot pointing jitter of the FEL that occurred between the reference measurement and the signal measurement. After calculating lineouts from Fig. 3a along the x axis, the resulting signal profiles were normalized to the corresponding reference profiles to account for the spatial FEL profile, as described in the Fig. 3c . This procedure yields the cross-correlation, , from equation (1), starting at and ending at , the transmission of the reference measurement. The temporal delay between FEL pulse and probe laser pulse was determined by the spatial position of the turning point of the cross-correlation curve. This position is independent from the FEL pointing jitter, because the deviation of the arrival time of the FEL wavefront can be neglected. For determining the FEL pulse duration, a nonlinear non-least square error optimization was used to fit calculated cross-correlations (equation (1)) to the measured transmission profiles ( Fig. 4 ). Calculations were carried out following the numerical procedure described above. For the optimization steps, Gaussian temporal FEL intensity profiles were assumed with varying pulse duration to calculate corresponding gating functions and the resulting cross-correlations. Exact knowledge about the temporal intensity profile of the near-infrared probe laser pulse, , is crucial to calculate the cross-correlations. This is of particular importance for FEL pulse durations approaching the probe laser pulse duration. Single-shot second-order autocorrelation measurements (device: Coherent SSA) were carried out to determine the laser pulse duration. Resolution of the measurement and error analysis The temporal resolution of the pulse duration measurement, Δ τ , is ultimately limited by the imaging resolution and the probe laser pulse duration. The imaging resolution was δ x =3.0 μm, corresponding to δ t =7 fs at δ =45° and δ t =10 fs at δ =14.2° (equation (7)). The pulse duration of the probe laser is uncertain within Δ τ Laser =±7 fs. This error arises from the resolution of the autocorrelator (8 fs per pixel) and the contribution from residual 3rd- and 4th-order dispersion from the grating compressor. We obtain the probe laser error contribution, Δ τ | Laser , by changing its pulse duration in the convolution integral (equation (6)) of the start-to-end simulation. The contribution to Δ τ results in Δ τ | Laser =±7 fs at 41.5 nm and Δ τ | Laser =±16 fs at 5.5 nm. For the presented measurements, further contributions to the error arise from statistical fluctuations of the data points (including imaging resolution) and the assumptions used in the mathematical model. These include also the deviation of the assumed plasma refractive index gradient from the unknown realistic free-electron profile and are estimated to be Δ τ | data =±12 fs at 41.5 nm and Δ τ | data =±10 fs at 5.5 nm, respectively. Thus, the overall error is estimated: giving Δ τ =±14 fs for the 41.5 nm and Δ τ =±19 fs for the 5.5-nm measurements. For reaching the ultimate temporal resolution, we propose applying a microscope objective with a higher numerical aperture (NA) to achieve diffraction-limited imaging. For example, with NA=0.8 and laser wavelength λ =500 nm, a spatial resolution of δ x =0.61 λ /NA=381 nm can be achieved, corresponding to δ t =1 fs. In combination with a sub-10-fs probe laser pulse, an overall resolution in the few-femtosecond regime is possible. How to cite this article: Riedel, R. et al . Single-shot pulse duration monitor for extreme ultraviolet and X-ray free-electron lasers. Nat. Commun. 4:1731 doi: 10.1038/ncomms2754 (2013).